Rice APC/CTEcontrols tillering by mediating the degradation of MONOCULM 1 Rice MONOCULM 1 ( MOC1 ) and its orthologues LS/LAS (lateral suppressor in tomato and Arabidopsis ) are key promoting factors of shoot branching and tillering in higher plants. However, the molecular mechanisms regulating MOC1/LS/LAS have remained elusive. Here we show that the rice tiller enhancer ( te ) mutant displays a drastically increased tiller number. We demonstrate that TE encodes a rice homologue of Cdh1, and that TE acts as an activator of the anaphase promoting complex/cyclosome (APC/C) complex. We show that TE coexpresses with MOC1 in the axil of leaves, where the APC/C TE complex mediates the degradation of MOC1 by the ubiquitin–26S proteasome pathway, and consequently downregulates the expression of the meristem identity gene Oryza sativa homeobox 1 , thus repressing axillary meristem initiation and formation. We conclude that besides having a conserved role in regulating cell cycle, APC/C TE has a unique function in regulating the plant-specific postembryonic shoot branching and tillering, which are major determinants of plant architecture and grain yield. Targeted protein degradation through the ubiquitin–proteasome system is a major regulatory mechanism of cell-cycle progression. Cdh1 (also known as Hct1 in budding yeast, Ste9 or Srw1 in fission yeast, Fzr in human and CCS52 in plants) is a substrate-recognition and -binding factor of the multimeric APC/C E3 ubiquitin ligase [1] . It is thought that Cdh1 activates APC/C in late mitosis and during G0/G1 by targeted degradation of key cell-cycle regulators (such as cyclins or inhibitors of cyclin-dependent kinases) by the 26S proteasome to promote mitotic exit, maintain G0/G1 phase and regulate the endocycle in animals [1] , [2] , [3] , [4] , [5] , [6] , [7] . Studies in Arabidopsis thaliana , legumes and tomato have also demonstrated that APC/C CCS52 regulates cell division, cell expansion, endocycle and root meristem maintenance [3] , [4] , [8] , [9] , [10] , [11] , [12] . However, other than mitotic cyclins, no substrates of APC/C CCS52 have been identified yet, and the regulatory mechanisms of APC/C CCS52 have remained essentially unknown in plants. Tillering and branching, the formation of lateral shoots, is an important determinant of plant architecture and crop yield [13] , [14] , and a complex process that is regulated by several genetic pathways [15] , [16] , [17] , [18] , [19] , [20] , [21] . The rice gene MOC1 and its orthologues LS / LAS encode transcriptional regulators of the GRAS family and are key promoting factors of tillering and branching in both monocot and dicot species [15] , [16] , [17] . Previous studies have shown that the LAS and MOC1 act upstream of SHOOT-MERISTEMLESS ( STM ) in Arabidopsis and OSH1 (the homologue of Knotted-1 in maize) during the initiation and establishment of AM [16] , [17] , [22] , [23] , [24] . However, the regulatory mechanisms of MOC1/LS/LAS have remained elusive. Here we report the identification of a tiller enhancer (te) mutant with many more tillers than wild-type rice. We show that TE is a rice homologue of Cdh1 , and it acts as an activator of APC/C to control rice tillering by mediating the degradation of MOC1 protein and, subsequently, reducing the expression of the meristem identity gene OSH1 . Our results provide new insights into the function and regulatory mechanisms of APC/C TE(Cdh1) E3 ligases in higher plants. The te mutant displays the pleiotropic phenotypes Rice-plant architecture is crucial for grain yield and is determined by tiller number and angle, plant height, panicle morphology, leaf structure and root systems [13] , [25] . To identify new regulators of rice architecture, we isolated the rice te mutant from a mutant pool [26] . te had a similar number of tillers as wild-type (WT) plants till the seventh leaf stage ( Fig. 1a ). However, by the heading stage, the total tiller number of te was about 3-fold that of WT, resulting from additional tillers produced on both low nodes and high nodes ( Fig. 1b–d ). In addition to increased tillers, the te mutant shows a dwarf phenotype with much shorter internodes II–V ( Fig. 1e,f ). Microscopy observation revealed that the shortening of te stem was mainly due to a reduction in cell number, as the cell sizes in internodes were largely comparable between WT and te ( Fig. 1g,h ). Moreover, the te mutant also displays a twisted flag leaf and panicle phenotype ( Fig. 1i–k ). 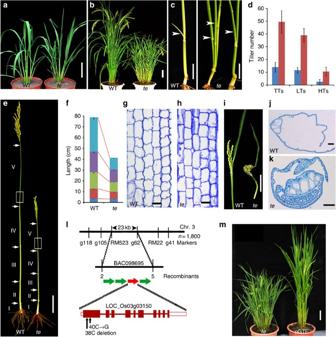Figure 1: Phenotype characterization oftemutant and map-based cloning ofTE. (a) Phenotype of WT andteplants at the seventh leaf stage. (b) Phenotype of WT andteplants at the heading stage. (c) WT produces un-elongated lateral bud (left panel, arrowhead) on the elongated upper internodes, whereastemutant produces additional tillers (right panel, arrowhead) from the elongated internodes. (d) Tiller number comparison between WT (blue) andte(red) plants at the heading stage. TTs, total tillers; LTs, lower node tillers; HTs, higher node tillers. LTs are the tillers outgrown from the un-elongated basal internodes. HTs are the tillers outgrown from the elongated internodes. (e) Stem structure of WT andte. (f) Internode length comparison between WT andte. I (light blue), II (purple), III (green), IV (red) and V (blue) indicate the first, the second, the third, fourth and fifth internode, respectively. (g,h) Longitudinal sections of the corresponding parts of the fifth internode (V) between WT (g) andte(h) (marked by white boxes ine). Scale bar, 50 μm. (i) The twisted panicle and flag leaf phenotype oftemutant. (j,k) Cross section images of flag leaf of WT (j) andtemutant (k) showing the highly twisted flag leaf structure oftemutant. (l) Mapping ofTElocus (LOC_Os03g03150) and the molecular lesions in thetemutant. (m) pGTE rescued thetemutant phenotype. Data are mean±s.d. (n=30 plants) ind,f. (a,b,c,e,i,m) Scale bar, 10 cm, (g,h) 50 μm and (j,k) 500 μm. Figure 1: Phenotype characterization of te mutant and map-based cloning of TE . ( a ) Phenotype of WT and te plants at the seventh leaf stage. ( b ) Phenotype of WT and te plants at the heading stage. ( c ) WT produces un-elongated lateral bud (left panel, arrowhead) on the elongated upper internodes, whereas te mutant produces additional tillers (right panel, arrowhead) from the elongated internodes. ( d ) Tiller number comparison between WT (blue) and te (red) plants at the heading stage. TTs, total tillers; LTs, lower node tillers; HTs, higher node tillers. LTs are the tillers outgrown from the un-elongated basal internodes. HTs are the tillers outgrown from the elongated internodes. ( e ) Stem structure of WT and te . ( f ) Internode length comparison between WT and te . I (light blue), II (purple), III (green), IV (red) and V (blue) indicate the first, the second, the third, fourth and fifth internode, respectively. ( g , h ) Longitudinal sections of the corresponding parts of the fifth internode (V) between WT ( g ) and te ( h ) (marked by white boxes in e ). Scale bar, 50 μm. ( i ) The twisted panicle and flag leaf phenotype of te mutant. ( j , k ) Cross section images of flag leaf of WT ( j ) and te mutant ( k ) showing the highly twisted flag leaf structure of te mutant. ( l ) Mapping of TE locus (LOC_Os03g03150) and the molecular lesions in the te mutant. ( m ) pGTE rescued the te mutant phenotype. Data are mean±s.d. ( n =30 plants) in d , f . ( a , b , c , e , i , m ) Scale bar, 10 cm, ( g , h ) 50 μm and ( j , k ) 500 μm. Full size image TE encodes a rice homologue of Cdh1 We used a map-based approach to place the TE locus within a 23-kb DNA region on the BAC098695 clone of chromosome 3, which contains four predicted genes. Two mutations, a deletion of nucleotide 38 (C) and a substitution of nucleotide 40 (C–G) downstream of the ATG initiation codon, were identified in the first exon of one of the predicted genes (LOC_Os03g03150) ( Fig. 1l ). These mutations result in a frame-shift and a 216-amino acid truncated protein product ( Supplementary Fig. S1 ). Genetic complementation showed that a genomic fragment containing the wild-type DNA (pGTE) completely rescued the te mutant phenotypes ( Fig. 1m ). We thus concluded that LOC_Os03g03150 corresponds to the TE gene. Sequence and phylogenetic analyses revealed that TE encodes a rice homologue of Cdh1 class proteins with a conserved WD-40 repeats domain and four motifs (C-box, CSM, RVL and IR) commonly found in other Cdh1 homologues ( Supplementary Figs S1 and S2 ). Quantitative reverse transcriptase–PCR analysis revealed that TE is widely expressed in roots, shoots, leaves and panicles ( Fig. 2a ). RNA in situ hybridization analysis demonstrated that TE is primarily expressed in the AM in axils from P1 to P5 leaf stage, shoot apical meristem and root meristem, and actively proliferative tissues such as young leaves ( Fig. 2b–e ). Thus, the expression pattern of TE is consistent with the phenotypes of te mutant. 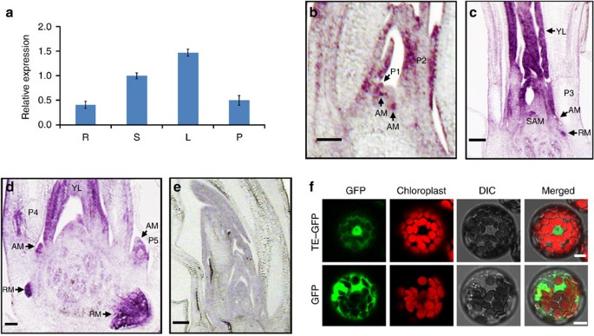Figure 2:TEexpression pattern and subcelluar localization of TE protein. (a) Quantitative RT–PCR analysis showing the relative expression levels ofTEin root (R), shoot (S), leaf (L) and panicle (P). Error bars represent s.e.m. (n=3). (b) RNAin situhybridization in longitudinal section showing thatTEis preferentially expressed in the AM in axils of P1 and P2 leaf, P1 leaf primordia and young leaves (YL) at P2 leaf stage. (c) RNAin situhybridization in longitudinal section showing thatTEis preferentially expressed in the shoot apical meristem (SAM), AM in axils of P3 leaf, root meristem (RM) and YL at P3 leaf stage. (d) RNAin situhybridization in longitudinal section showing thatTEis preferentially expressed in the AM in axils of P4 leaf and P5 leaf, RM and YL at P4 leaf stage. (e) The sense probe ofTEwas used as a negative control. (f) TE–GFP fusion protein is predominantly localized to the nuclei ofArabidopsisprotoplasts (upper images); GFP protein itself is distributed throughout the cytoplasm ofArabidopsisprotoplasts (lower images). (b–e) Scale bar, 100 μm and (f) 7.5 μm. Figure 2: TE expression pattern and subcelluar localization of TE protein. ( a ) Quantitative RT–PCR analysis showing the relative expression levels of TE in root (R), shoot (S), leaf (L) and panicle (P). Error bars represent s.e.m. ( n =3). ( b ) RNA in situ hybridization in longitudinal section showing that TE is preferentially expressed in the AM in axils of P1 and P2 leaf, P1 leaf primordia and young leaves (YL) at P2 leaf stage. ( c ) RNA in situ hybridization in longitudinal section showing that TE is preferentially expressed in the shoot apical meristem (SAM), AM in axils of P3 leaf, root meristem (RM) and YL at P3 leaf stage. ( d ) RNA in situ hybridization in longitudinal section showing that TE is preferentially expressed in the AM in axils of P4 leaf and P5 leaf, RM and YL at P4 leaf stage. ( e ) The sense probe of TE was used as a negative control. ( f ) TE–GFP fusion protein is predominantly localized to the nuclei of Arabidopsis protoplasts (upper images); GFP protein itself is distributed throughout the cytoplasm of Arabidopsis protoplasts (lower images). ( b–e ) Scale bar, 100 μm and ( f ) 7.5 μm. Full size image As reported for other Cdh1 homologues such as AtCCS52A1 and AtCCS52A2 [8] , transient expression analysis in Arabidopsis protoplasts revealed that the TE–GFP fusion protein is predominantly targeted to the nucleus ( Fig. 2f ). Overexpression of TE in Schizosaccharomyces pombe inhibited cell division and caused cell enlargement ( Fig. 3a,b ). Consistent with this observation, flow cytometry and 4′,6-diamidino-2-phenylindole staining analyses showed that some cells in the te flag leaves had 4C DNA content and were binucleated compared with WT, suggesting a delay in mitotic exit in some te leaf cells ( Fig. 3c–f ). Notably, more binucleated cells have been observed in mice Fzr1 −/− mouse embryonic fibroblasts ( Cdh1 -deficient cells) because of delayed mitotic exit [27] . Taken together, these results support the notion that TE has an evolutionarily conserved role in cell-cycle regulation [2] , [27] , [28] . 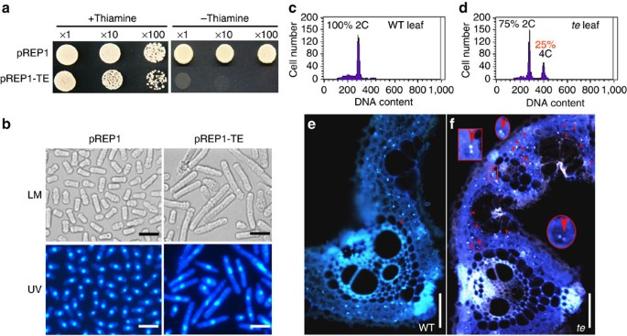Figure 3: Conserved role ofTEin cell-cycle regulation. (a) Growth ofS. pombetransformed with the empty vector pREP1 and pREP1-TE in the presence (+thiamine, the expression ofTEis repressed in the presence of thiamine) or absence of thiamine (−thiamine, the expression ofTEis induced in the absence of thiamine). (b) The observation ofS. pombecells under light microscopy and 4′,6-diamidino-2-phenylindole (DAPI)-stained cells under UV light showing theS. pombecells transformed with pREP1-TE in the absence of thiamine became much larger and longer concomitant with bigger nuclei compared with pREP1. LM, light microscopy; UV, observation of DAPI-stained cells under UV light. (c,d) Flow cytometry analysis showing that some (about 25%) flag leaf cells oftemutant (d) have 4C DNA content compared with WT (c). (e,f) Microscopy images of transverse sections (stained with DAPI) showing that the flag leaves ofte(f) have more cells with two nuclei (indicated by arrowheads) compared with WT flag leaves (e). The inset magnified parts infshowing two nuclei in one cell. (b) Scale bar, 10 μm and (e,f) 50 μm. Figure 3: Conserved role of TE in cell-cycle regulation. ( a ) Growth of S. pombe transformed with the empty vector pREP1 and pREP1-TE in the presence (+thiamine, the expression of TE is repressed in the presence of thiamine) or absence of thiamine (−thiamine, the expression of TE is induced in the absence of thiamine). ( b ) The observation of S. pombe cells under light microscopy and 4′,6-diamidino-2-phenylindole (DAPI)-stained cells under UV light showing the S. pombe cells transformed with pREP1-TE in the absence of thiamine became much larger and longer concomitant with bigger nuclei compared with pREP1. LM, light microscopy; UV, observation of DAPI-stained cells under UV light. ( c , d ) Flow cytometry analysis showing that some (about 25%) flag leaf cells of te mutant ( d ) have 4C DNA content compared with WT ( c ). ( e , f ) Microscopy images of transverse sections (stained with DAPI) showing that the flag leaves of te ( f ) have more cells with two nuclei (indicated by arrowheads) compared with WT flag leaves ( e ). The inset magnified parts in f showing two nuclei in one cell. ( b ) Scale bar, 10 μm and ( e,f ) 50 μm. Full size image TE physically interacts with MOC1 and OsCDC27 It has been reported previously that Cdh1 mainly recognizes the D-box (RxxLxxxxN/D/E) and KEN-box in the amino-terminal region of its substrates to target them for ubiquitination and degradation by the 26S proteasome [1] , [7] . The enhanced tillering phenotype in the loss-of-function te mutant suggests that TE could participate in targeted degradation of a positive regulator(s) of tillering. Through extensive analysis of known positive regulators of tillering and branching, we identified a typical D-box in the N-terminal region of the MOC1/LS/LAS protein ( Supplementary Fig. S3a ). Previous studies have reported a loss-of-function moc1 mutant that has dramatically reduced tiller number, whereas MOC1- overexpressing lines have increased tiller number [17] . Thus, we tested whether TE physically interacts with MOC1. A yeast two-hybrid assay showed that TE interacted with MOC1, but not with MOC1-d (deletion of 107 amino acids in the N-terminal region) or MOC1-m (in which the typical D-box was mutated) ( Fig. 4a ). In addition, an in vitro pull-down assay showed that MBP–TE protein but not the MBP control pulled down MOC1 protein from the total protein extracts of WT rice plants ( Fig. 4b ). Moreover, biomolecular fluorescence complementation (BiFC) assay showed that TE interacted with MOC1 in Nicotiana benthamiana leaf cells ( Fig. 4c ). These results suggest that TE directly interacts with MOC1 and that the D-box in the N-terminal region of MOC1 is required for its physical interaction with TE. 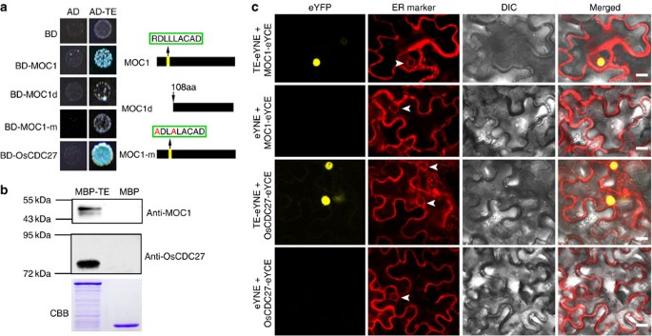Figure 4: TE physically interacts with MOC1 and OsCDC27. (a) Yeast two-hybrid assay showing that TE interacts with MOC1 and OsCDC27, but not with MOC1d and MOC1-m. The protein structure of MOC1 and MOC1d and the amino-acid substitutions in MOC1-m are shown on the right. (b)In vitropull-down assay showing that MBP–TE, but not MBP itself, pulled down MOC1 (upper image) and OsCDC27 (middle image) from plant extracts. Coomassie blue staining (CBB) showing that roughly equal amounts of purified MBP-TE and MBP proteins were used in the pull-down assay (lower image). (c) BiFC assay showing that TE can interact with MOC1 and OsCDC27 in the nuclei of leaf cells ofN. benthamiana. The signals of eYFP were not detected in the corresponding negative controls. White arrowheads indicate the nuclear membrane. Scale bar, 20 μm. Figure 4: TE physically interacts with MOC1 and OsCDC27. ( a ) Yeast two-hybrid assay showing that TE interacts with MOC1 and OsCDC27, but not with MOC1d and MOC1-m. The protein structure of MOC1 and MOC1d and the amino-acid substitutions in MOC1-m are shown on the right. ( b ) In vitro pull-down assay showing that MBP–TE, but not MBP itself, pulled down MOC1 (upper image) and OsCDC27 (middle image) from plant extracts. Coomassie blue staining (CBB) showing that roughly equal amounts of purified MBP-TE and MBP proteins were used in the pull-down assay (lower image). ( c ) BiFC assay showing that TE can interact with MOC1 and OsCDC27 in the nuclei of leaf cells of N. benthamiana . The signals of eYFP were not detected in the corresponding negative controls. White arrowheads indicate the nuclear membrane. Scale bar, 20 μm. Full size image Cdh1 activates the activity of APC/C Cdh1 E3 ubiquitin ligase by coupling to the CDC27 subunit of the APC/C complex [1] , [7] . The rice genome contains a single CDC27 gene, OsCDC27 ( Supplementary Fig. S3b,c ). We confirmed that TE indeed physically interacts with OsCDC27 using yeast two-hybrid, in vitro pull-down and BiFC assays ( Fig. 4a–c ). These results support the notion that TE acts as an activator of APC/C E3 ubiquitin ligase by directly coupling to the OsCDC27 subunit of the APC/C complex. TE mediates the degradation of MOC1 We next conducted a series of biochemical experiments to test whether TE mediates the proteolysis of MOC1. An in vitro ubiquitination assay showed that MOC1 was polyubiquitinated by the total protein extracts of WT plants, but not by extracts of te plants ( Fig. 5a , Supplementary Fig. S4 ), indicating that TE is required for MOC1's ubiquitination. In addition, a cell-free degradation study showed that purified recombinant MBP–MOC1 protein, but not the MBP–MOC1-m protein and MBP control, was rapidly degraded by the total protein extracts of WT plants, but not by extracts of te plants ( Fig. 5b ). Moreover, MG132, a specific inhibitor of the 26S proteasome, blocked the degradation of MBP–MOC1 in the total protein extracts ( Fig. 5b ). Further, MOC1 protein level was markedly higher in te plants compared with WT plants ( Fig. 5c ) whereas TE -overexpression lines ( TE -OE) had reduced MOC1 accumulation and reduced tiller number ( Fig. 5d–f ). Taken together, these results support the view that TE regulates tillering in rice by mediating the degradation of MOC1 by the ubiquitin–26S proteasome pathway. 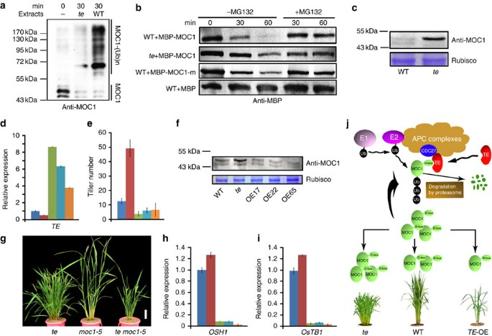Figure 5: TE mediates the degradation of MOC1 and it acts upstream of MOC1. (a)In vitroubiquitination assay showing that MOC1 is ubiquitinated by WT plant extracts but not byteplant extracts. (b) Cell-free degradation assay showing that MBP-MOC1, but not MBP-MOC1-m and MBP, was degraded in WT plant extracts after 60 min incubation, whereas MBP-MOC1 remained relatively stable inteplant extracts. The degradation of MBP-MOC1 by plant extracts was blocked in the presence of 40 μM MG132 (+MG132). (c) Western blot analysis showing that MOC1 protein accumulated to a higher level in theteplants compared with WT (top). Rubisco strips showing a roughly equal loading of total proteins (bottom). (d) Quantitative RT–PCR assay showing that the expression level ofTEis dramatically upregulated in OE17 (green), OE22 (light blue) and OE65 (orange), compared with WT (blue) orte(red). (e) OE17 (green), OE22 (light blue) and OE65 (orange) had reduced tiller numbers in comparison with WT (blue) orte(red). Data are mean±s.d. (n=15 plants). (f) Western blot analysis showing that there was less MOC1 protein in theTE-OE lines compared with WT andte(top). Rubisco strips showing the roughly equal loading of total proteins (bottom). (g) Thete moc1-5double mutant have reduced tiller number as themoc1-5parent. Scale bar,10 cm. (h,i) Quantitative RT–PCR assay showing that the expression levels ofOSH1andOsTB1were drastically reduced in OE17 (green), OE22 (light blue) and OE65 (orange) transgenic lines, but slightly increased inte(red) mutant, in comparison with WT (blue). (j) A model showing that TE activates the APC/C E3 ubiquitin ligase activity and targets MOC1 for degradation through interacting with the D-box, and consequently represses tillering. Error bars represent s.e.m. ind,h,i(n=3). Figure 5: TE mediates the degradation of MOC1 and it acts upstream of MOC1. ( a ) In vitro ubiquitination assay showing that MOC1 is ubiquitinated by WT plant extracts but not by te plant extracts. ( b ) Cell-free degradation assay showing that MBP-MOC1, but not MBP-MOC1-m and MBP, was degraded in WT plant extracts after 60 min incubation, whereas MBP-MOC1 remained relatively stable in te plant extracts. The degradation of MBP-MOC1 by plant extracts was blocked in the presence of 40 μM MG132 (+MG132). ( c ) Western blot analysis showing that MOC1 protein accumulated to a higher level in the te plants compared with WT (top). Rubisco strips showing a roughly equal loading of total proteins (bottom). ( d ) Quantitative RT–PCR assay showing that the expression level of TE is dramatically upregulated in OE17 (green), OE22 (light blue) and OE65 (orange), compared with WT (blue) or te (red). ( e ) OE17 (green), OE22 (light blue) and OE65 (orange) had reduced tiller numbers in comparison with WT (blue) or te (red). Data are mean±s.d. ( n =15 plants). ( f ) Western blot analysis showing that there was less MOC1 protein in the TE -OE lines compared with WT and te (top). Rubisco strips showing the roughly equal loading of total proteins (bottom). ( g ) The te moc1-5 double mutant have reduced tiller number as the moc1-5 parent. Scale bar,10 cm. ( h , i ) Quantitative RT–PCR assay showing that the expression levels of OSH1 and OsTB1 were drastically reduced in OE17 (green), OE22 (light blue) and OE65 (orange) transgenic lines, but slightly increased in te (red) mutant, in comparison with WT (blue). ( j ) A model showing that TE activates the APC/C E3 ubiquitin ligase activity and targets MOC1 for degradation through interacting with the D-box, and consequently represses tillering. Error bars represent s.e.m. in d , h , i ( n =3). Full size image To further determine the genetic interaction between TE and MOC1, we isolated a new allele of moc1 , termed moc1-5 , and constructed the te moc1-5 double mutant. Map-based cloning and sequence analysis identified a deletion of nucleotide 38 (C) downstream of the ATG initiation codon of the MOC1 gene (LOC_Os06g40780) in the moc1-5 mutant ( Supplementary Fig. S5a ), leading to a frame-shift and a 267-amino acid truncated protein product. Western blot analysis confirmed the absence of the MOC1 protein in moc1-5 mutant ( Supplementary Fig. S5b ). Like the moc1-5 mutant, the te moc1-5 double mutant had significantly reduced number of tillers ( Fig. 5g ), suggesting that MOC1 acts downstream of TE in control of tillering. Consistent with this, the expression of OSH1 [24] , [29] , [30] (a key meristem identity gene) and OsTB1 [31] (a rice homologue of maize TB1 [32] ) was markedly lower in our TE -OE lines as in moc1 mutant [17] ( Fig. 5h,i ), further supporting the notion that TE and MOC1 act in the same genetic pathway in control of tillering. Tillering or formation of shoot branches is a postembryonic developmental process unique to higher plants. The shoot branches originate from AMs that are produced in the axils of the leaves. Several key regulators involved in AM formation have been identified in plants, including REVOLUTA [33] , LAS [16] and Regulator of Axillary Meristem [34] in Arabidopsis , LS [15] , [16] and Blind in tomato [35] , Barren Stalk1 (BA1) [19] in maize, MOC1 [17] , Lax Panicle1 [18] , [36] and Lax Panicle2 [21] in rice. Here, we have identified a new negative regulator of tillering in rice, TE, and demonstrated that it acts as an activator of APC/C E3 ubiquitin ligase. We further showed that TE has a conserved role in cell-cycle regulation and that it regulates rice tillering by mediating the degradation of MOC1 ( Fig. 5j ), and consequently downregulates the expression of the meristem identity gene OSH1 ( Fig. 5h ), thus repressing AM initiation and formation. These results indicate that plants and animals could use conserved cell-cycle machineries to regulate distinct developmental processes. To our knowledge, MOC1 is the first reported substrate of APC/C CCS52 that is not a mitotic cyclins in plants, and its orthologues in tomato (LS) and Arabidopsis (LAS) have also been shown to have a similar role in regulating lateral branching (shoot and panicle branching) [15] , [16] . In addition, the putative orthologues of TE (CCS52 proteins in Arabidopsis, maize, tomato and legume) [4] , [8] , [12] , [37] and OSH1 (KN1 in maize and STM in Arabidopsis ) [22] , [23] could be identified in both monocot and dicot species. Further, previous studies have shown that LAS acts upstream of REVOLUTA , which is needed to activate the expression of STM in Arabidopsis [16] , [33] . These results together suggest that a conserved genetic pathway (TE(CCS52A)–MOC1(LAS)– OSH1 ( STM )) likely operates in both monocots and dicots to control tillering and shoot branching. The observed overlap of TE and MOC1 expression in the axil from P2 to P3 leaf stage ( Fig. 2b–d , refs 17 and 36 ) suggests that a link probably exists between the levels of TE and MOC1 proteins to the state of stem cell-like cells in the axils from P1 to P3 leaf stage. We speculate that TE might act to maintain these stem cell-like cells in a mitotically inactive and indeterminate state through targeted proteolysis of MOC1, a key AM-initiation-promoting factor (refs 17 17 and 36 ). In further support of this notion, we have demonstrated that TE -OE lines have much fewer tillers concomitant with reduced level of MOC1 protein accumulation, whereas the loss-of-function te mutants have much more tillers concomitant with the elevated level of MOC1 protein accumulation ( Fig. 5 ). In addition to cell-cycle regulation, APC/C Cdh1 has been reported to have important roles in regulating hematopoiesis, neurogenesis, lens development, myogenesis, genomic stability and tumour suppression by targeted degradation of specific key regulators of these developmental processes in animals [2] , [28] , [38] . APC/C CCS52 has also been shown to regulate root development in plants [8] . In this study, we found that the te mutant displayed a pleiotropic phenotype, including shortened stem and flag leaves, twisted flag leaves and panicles ( Fig. 1e–k ), suggesting that, as in animals, APC/C CCS52A also has important roles in regulating a variety of developmental processes in plants. Further investigation of the detailed mechanisms of APC/C TE(CCS52A) regulating plant morphogenesis, and the functional relationship of the (TE(CCS52A)-MOC1(LAS)- OSH1 ( STM )) pathway with other developmental pathways regulating branching pattern (such as the Lax Panicle1/BA1 pathway [18] , [19] , [36] and the MAX/RMS/D pathway [39] ), may provide new strategies for genetic improvement of crop architecture to optimize grain yield. Plant materials The te mutant was identified from the F 4 offsprings of pollen culture plants derived from the tetraploid hybrid H5409 (H2088xH3811) [26] . The normal offspring of pollen culture plants, with a nearly identical genetic background to te , was viewed as the wild type (WT) of te in this study. Genetic analysis showed that the twisted leaf phenotype of te is controlled by a single recessive nuclear locus, TE . To map the TE locus, we generated an F 2 mapping population derived from a cross between the te and the cultivar Zhenshan 97B. Map-based cloning of TE The TE locus was mapped to a 23-kb region between the simple sequence repeat marker RM523 and the InDel marker g62 on chromosome 3 using 1,800 F 2 mutant plants with additionally molecular markers developed in this work ( Supplementary Table S1 ). The cDNA of the candidate gene, LOC_Os03g03150, was amplified from both te and WT using primers (Rt-1F 5′-ACCTTCCTCTCCTCTCCTCCC-3′ and Rt-1R 5′-TCAGTGTTTGCCATCTTCGCT-3′), and the PCR products were confirmed by sequencing. Construction of te moc1-5 double mutant The moc1-5 mutant was isolated from a population of Nipponbare treated by 60 Co-γ irradiation. The mutation locus was mapped with markers developed in this study ( Supplementary Table S2 ). The te moc1-5 double mutants were identified from F 2 offsprings of the hybrids between te and moc1-5 mutant. Complementation test and overexpression of TE in te plants A 6.2-kb genomic DNA fragment (consisting of a 1.2-kb upstream sequence, the entire TE gene including ten exons and nine introns, and a 1.1-kb downstream region) was amplified using primers pGR-3F (5′-TGAATCTTACTCTTCTATATATTGCCTCAC-3′) and pGR-4R (5′-GGATCCCATAACCTTATTTATTTTTCTAGT-3′), and the PCR product was inserted into the binary vector pCAMBIA1305.1 to generate the transformation plasmid pGTE. The 1.8-kb cDNA sequence of TE was amplified using primers RT-2LF (5′-ATCCCCAAATCTCTCGCCCCCACCCA-3′) and RT-2LR (5′-TCGCTCCTACAAAGCCAATGAATAAA-3′), and the PCR fragment was inserted into the downstream of the ubiquitin promoter in the vector pCUBi 1390, resulting in plasmid pUBi ∷ TE. The te was transformed with Agrobacterium tumefaciens strain EHA105 harbouring the plasmid pGTE or pUBi ∷ TE. RNA in situ hybridization Shoot apexes of rice seedlings at the third and fourth leaf stages were fixed with an formalin acetic-acid alcohol (RNase-free) fixative solution at 4 °C overnight, followed by a series of dehydration steps and then embedded in paraffin (Paraplast Plus, Sigma). RNA in situ hybridization was performed as described previously [40] . The 5′ end of TE was amplified with primers pf2 (5′-ACTGAGATGTGGAGCGAAGATGG-3′) and pr2 (5′-TTGACATAGATCAGTACAAAGTTG-3′) and cloned into the pGEM-T Easy vector (Promega). Digoxigenin-labelled probes were prepared from linearized templates amplified from the pGEM-T plasmid containing the 5′ end of TE using primer Yt7 (5′-CCCAGTCACGACGTTGTAAA-3′) and Ysp6 (5′-CACACAGGAAACAGCTATGAC-3′). Digoxigenin-labelled RNA probes were prepared using a DIG Northern Starter Kit (Cat. No. 2039672, Roche) following the instructions of manufacturer. The slides were observed under bright field with a microscope (Leica DM5000B) and photographed using a camera (Leica DFC490). Subcellular localization A 1,569-bp coding sequence of TE was amplified with the primer 52aXF (5′-CTAGATCTCGAGATGGATCACCACCACCACCACCTG-3′) and 52aSR (5′-CTAGACTAGTCGGATGTAGCTCCTAACAAATGATG-3′), and the PCR product was inserted into the Xho I/ Spe I sites of the PA7 vector, to fuse to the upstream of GFP, resulting in the TE–GFP fusion protein-expressing plasmid PA7-TE, and then transformed into Arabidopsis protoplasts, as reported previously [41] . PA7 plasmid was used as the control. Flow cytometry About 30 flag leaves were chopped in 10 ml of a cold nuclear isolation buffer (10 mM MgSO 4 , 50 mM KCl, 5 mM hepes (4-(2-hydroxyethyl) piperazine-1-ethanesulfonic acid), 3 mM dithiothreitol, pH 8.0. Triton X-100 at a final concentration of 0.25% before use). The crude extract with isolated cells was filtered (48 μm), then stained with 2.5 μg ml −1 4′,6-diamidino-2-phenylindole (DAPI, Roche) and immediately analysed on an FACStar Plus cytometer (Becton Dickinson). Overexpression of TE in Schizosaccharomyces pombe The coding sequence of TE was amplified using primer 52aNF (5′-GGAATTCCATATGATGGATCACCACCACCACCACCTG-3′) and 52aBR (5′-CTAGGAAGATCTTCACCGGATGTAGCTCCTAACAAATG-3′), and the PCR product was cloned into the pREP1 vector and verified by sequencing. In the absence of thiamine (-thiamine), overexpression of TE was induced in S. pombe as reported [3] . Construction of protein expression plasmids MOC1 and TE were amplified with the primers shown in Supplementary Table S3 , and the PCR products were cloned into the pMAL-C2x vector (NEB), resulting in the plasmids pMAL-C2x ∷ MBP-MOC1 and pMAL-C2x ∷ MBP-Te. The D-box of MOC1 was mutated using a Phusion® Site-Directed Mutagenesis Kit (NEB) with the primers listed in Supplementary Table S3 . In vitro pull-down assay The seedlings of wild type were planted in the pots and grown in a climate chamber (HP1500GS, Ruihua) with a 14.5-h light (30 °C) −9.5 h darkness (25 °C) photocycle. Total proteins were subsequently extracted in a degradation buffer [42] . The total protein concentration was determined by the Bio-Rad protein assay. For pull-down assay, roughly equal amounts of purified MBP and MBP–TE fusion proteins (about 1 μg) were affixed to Amylose Resin (NEB), and incubated in 400 μl of plant extract (containing 1.6 mg total proteins) in the presence of 42 μM MG132 gently shaken at 28 °C for 30 min. The pull-down analyses were performed as reported [43] , [44] and detected with anti-MOC1 or anti-OsCDC27 antibodies at 1:200 dilution. The horseradish peroxidase (HRP)-conjugated anti-rabbit IG (H+L) (1:5,000 dilution, MBL) was used as the second antibody. The western blots were developed with enhanced chemiluminescence (ECL) reagent (GE Healthcare). Cell-free degradation assay The total protein extracts were prepared as in the pull-down assay from te and WT seedlings, and were adjusted to equal concentration in the degradation buffer [42] . Then MG132 (Calbiochem) was selectively added to various in vitro degradation assays as indicated. For degradation of purified MBP, MBP-MOC1 and MBP-MOC1-m proteins, equal amounts of these purified proteins (about 500 ng) were incubated in 50 μl of rice total-protein extract (containing about 200 μg total proteins) at 28 °C for each assay. For mock controls, an equal amount of solvent for each drug was used. The extracts were incubated at 28 °C, and the samples were taken at the indicated intervals for determination of MBP, MBP-MOC1 and MBP-MOC1-m protein abundance by western blots with the HRP-conjugated Anti-MBP monoclonal antibody at 1:5,000 dilution (E8038L, NEB). The western blots were developed with ECL reagent (GE Healthcare). Yeast two-hybrid assay The coding sequences of TE , OsCDC27 , MOC1 , MOC1d and MOC1-m were amplified using gene-specific primers ( Supplementary Table S4 ). TE was inserted into the pGADT7 vector (Clonetech), and MOC1 , MOC1d , MOC1-m and OsCDC27 were inserted into the pGBKT7 vector (Clonetech), respectively. The yeast two-hybrid assay was performed following the manufacturer's instructions. Antibody preparation and western blot analysis MOC1 CDS was inserted into the pET32a vector. Purified His-MOC1 fusion protein was injected into rabbits to produce polyclonal antibodies of MOC1. Western blots were performed using antiserum against MOC1 and visualized by an enhanced HRP-DAB substrate kit (PA110, TIANGEN). For OsCDC27, the polypeptide FNQSSDSVPRRSAR was synthesized, and conjugated with keyhole limpet hemocyanin (KLH) to form KLH-FNQSSDSVPRRSAR. Subsequently, the conjugates were injected into rabbits to produce polyclonal antibodies against OsCDC27. In vitro ubiquitination assay The purified MBP–MOC1 protein bound to the Amylose Resin (NEB) was incubated at 28 °C with equal amounts of rice seedling crude extract in a buffer containing 25 mM Tris–HCl pH 7.5, 10 mM MgCl 2 , 5 mM dithiothreitol, 10 mM NaCl, 10 mM adenosine triphosphate and 40 μM MG132. After incubation at 28 °C for the intervals as indicated, the MBP–MOC1 and MBP–MOC1-(Ub)n fusion proteins were cleaved at room temperature by Factor Xa (NEB), following the manufacturer's instruction. The supernatant containing MOC1 or MOC1-(Ub)n was added with SDS–PAGE-loading buffer, then loaded on SDS–PAGE gel and western blots were performed using antibodies against MOC1 or antibodies against polyubiquitin (Beijing Protein Innovation, http://www.proteomics.org.cn/ ) at 1:200 dilution. The HRP-conjugated anti-rabbit IG (H+L) (1:5,000 dilution, MBL) was used as the second antibody. The western blots were developed with ECL reagent (GE Healthcare). Quantitative RT–PCR analysis RNA was extracted from frozen samples using the RNAprep Pure Plant Kit (Tiagen) following the manufacturer's instructions. Quantitative RT–PCRs were performed by a SYBR Premix Ex Taq™ RT–PCR kit (Takara) following the manufacturer's instructions with the primers listed in Supplementary Table S5 . BiFC assay CDS of TE was amplified with primer 52aSF (5′-GGAATTCACTAGTATGGATCACCACCACCACCACCTG-3′) and 52aKR (5′-CTAGGAGGTACCCCGGATGTAGCTCCTAACAAATG-3′), then cloned into the Spe I/ Kpn I sites of the vector pSPYNE173 (eYNE) [45] to form the TE-eYNE plasmid. CDS of MOC1 was amplified with primer MOC1BF (5′-AGATTCGGATCCATGCTCCGGTCACTCCACTCCTC-3′) and MOC1KR (5′-CTAGGAGGTACCCGACGACGACGGCTGC-3′), then cloned into the Bam HI/Kpn I sites of the vector pSPYCE(M) (eYCE) [45] to form the MOC1-eYCE plasmid. CDS of OsCDC27 was amplified with primer CDC27SF (5′-GGAATTCACTAGTATGGAAACCCTAATGGTGGACCG-3′) and CDC27XR (5′-CTAGGACTCGAGAATCTCATCATCATCATCATCATCATCC-3′), then cloned into the Spe I/ Xho I sites of the vector pSPYCE(M) to form the CDC27-eYCE plasmid. For transient expression, A. tumefaciens strain AH109 carrying the BiFC constructs were used together with the p19 strain [46] and ER marker, mCherry ER-rk CD3-959 [47] , for infiltration of 5–6-week-old N. benthamiana leaves, as described in Waadt and Kudla [48] . Infiltrated leaves were observed 48–72 h after infiltration using a laser confocal scanning microscope (ZEISS Microsystems LSM 700, http://www.zeiss.com.cn/microscopy ). The eYFP and mCherry fluorescent signals from the expressed fusion constructs were monitored sequentially. The excitation and detection wavelengths for eYFP and mCherry were 514 and 587 nm for excitation, and 527 and 610 nm for detection, respectively. How to cite this article: Lin, Q. et al . Rice APC/C TE controls tillering by mediating the degradation of MONOCULM 1. Nat. Commun. 3:752 doi: 10.1038/ncomms1716 (2012).